Structure of a bacterial α2-macroglobulin reveals mimicry of eukaryotic innate immunity Alpha-2-macroglobulins (A2Ms) are plasma proteins that trap and inhibit a broad range of proteases and are major components of the eukaryotic innate immune system. Surprisingly, A2M-like proteins were identified in pathogenically invasive bacteria and species that colonize higher eukaryotes. Bacterial A2Ms are located in the periplasm where they are believed to provide protection to the cell by trapping external proteases through a covalent interaction with an activated thioester. Here we report the crystal structures and characterization of Salmonella enterica ser. Typhimurium A2M in different states of thioester activation. The structures reveal thirteen domains whose arrangement displays high similarity to proteins involved in eukaryotic immune defence. A structural lock mechanism maintains the stability of the buried thioester, a requirement for its protease-trapping activity. These findings indicate that bacteria have developed a rudimentary innate immune system whose mechanism mimics that of eukaryotes. Alpha-2-macroglobulins (A2Ms) are highly conserved, broad-spectrum protease inhibitors that play key roles in eukaryotic innate immunity; their main functions include clearing pathogenic or parasitic proteases from circulation. A2Ms are composed of ~180 kDa subunits that generally associate into homotetrameric or homodimeric forms [1] , [2] , [3] . Each A2M monomer is characterized by a highly reactive thioester bond as well as a bait region whose sequence is recognized by a variety of proteases. Protease entrapment occurs through a ‘Venus flytrap mechanism’ [4] , [5] involving proteolytic cleavage of the recognized bait region, followed by a large conformational change that blocks the target protease within a cage-like complex. Exposure of the highly reactive thioester site (CXEQ), which associates covalently to the protease, prevents its escape. This conformational modification also exposes a C-terminal, receptor-binding region that subsequently binds to the low-density lipoprotein receptor on target cells, allowing clearance of the complex [6] . It is of note that the thioester site can be inactivated by reaction with small nucleophiles such as methylamine, ethylamine or ammonia [3] , [7] , [8] , [9] . Following reaction with methylamine, A2M adopts a conformation that resembles the protease-reacted form [10] , [11] . A2Ms and the components of the complement system, such as factors C3 and C4, form a superfamily of proteins that are structurally similar and evolutionarily related [2] , [12] . Also part of this superfamily, but much less well characterized, are pregnancy zone protein, CD109, CPAMD8 and A2ML1 (refs 13 , 14 , 15 , 16 ). Most of the proteins in the superfamily carry the CXEQ thioester motif, attesting to the fact that the biological activity of all members is linked to their capacity to generate a covalent bond with their target molecules. C3, for example, is a multidomain, two-chain, 187-kDa molecule whose activation by proteolysis is a pivotal step of the complement cascade. Its CXEQ motif, which is harboured within the thioester-containing domain (TED), becomes exposed after a large conformational change and is then able to associate covalently to the cell wall of antigens during opsonization. Interestingly, insect thioester-containing protein (TEP), which is found in the haemolymph and functions in the innate immune system of insects, appears to have similar features to both A2M and complement C3, also utilizing a thioester site for opsonization [17] , [18] . A commonality observed between these proteins is thus a role in immunological function and the exploitation of the thioester to form covalent linkages. Recently, a 4.3-Å resolution structure of methylamine-treated human A2M [5] in tetrameric form revealed the overall, multidomain fold of the protein, but atomic details were not described. In addition, electron microscopy structures have provided some insight into the conformational change undergone by eukaryotic A2M in the protease-trapping process [10] , [19] , [20] , but there are no crystal structures of A2M in the native or protease-activated forms. Insight into the mechanism of target protease trapping has been obtained from crystal structures of components of the complement system and mosquito TEP1, which provide details about the architecture of the A2M/complement/TEP superfamily and the domain rearrangements that are required for the activation of these proteins [17] , [21] , [22] , [23] , [24] , [25] , [26] , [27] , but these details remain specific to proteins involved in complement activation. Thus, despite the central importance of A2Ms in innate immunity, detailed structural characterization of an A2M is still lacking. In spite of the fact that molecules of the A2M/complement/TEP superfamily were believed to be limited to metazoans, genomic analyses revealed that genes for A2M-like proteins also exist in several bacterial species, many of which are pathogenic or are common colonizers of higher eukaryotes [28] . Two forms of A2M-like proteins were identified, only one of which contains the hallmark CXEQ thioester motif. Some bacteria, such as Escherichia coli , carry both forms of A2M, while others, such as Salmonella enterica or Pseudomonas aeruginosa , carry only one form. P. aeruginosa expresses a single A2M variant that does not carry an CXEQ motif in its sequence; nevertheless, its expression has been associated to the coexpression of genes encoding elements of the type VI secretion system as well as biofilm formation [29] , [30] , indicating a strong link with pathogenesis. Interestingly, in a number of bacteria, including S. enterica ser. Typhimurium ( S. typhimurium ), the gene for the thioester-containing form is often found adjacent to the one encoding Penicillin-Binding Protein 1c (PBP1c). Since PBPs are involved in peptidoglycan synthesis, CXEQ-carrying bacterial A2Ms were hypothesized to work conjunctively with PBP1c as a periplasmic defence system [28] . In the event of a cell wall breach, the bacterial A2M would inhibit the antibacterial proteases, while PBP1c would repair the cell wall by catalysing the polymerization of glycan chains within the damaged peptidolgycan [28] , [31] . Biochemical characterization of the thioester-containing E. coli A2M (ECAM) showed that, unlike human A2M, it is a monomer, and is anchored to the inner membrane, thus being localized in the periplasmic space [32] , [33] . ECAM is capable of binding proteases and hindering their access to substrates, which supports the potentially defensive role of A2M-like proteins in bacteria. To gain insight into the potential function of A2Ms in bacterial defence, their mechanism of action and their structure in atomic detail, we solved the crystal structures of S. typhimurium A2M (Sa-A2M) in native, inactivated and mutant forms. These structures provide validation of the bacterial A2Ms as members of the A2M/complement/TEP superfamily of proteins. Reaction of Sa-A2M with methylamine generated local conformational changes within the thioester site region, allowing the identification of an amino-acid ‘locking mechanism’ that prevents thioester accessibility in the absence of substrate. In addition, an engineered variant of Sa-A2M harbouring a bait region modified to recognize tobacco etch virus (TEV) protease could be shown to covalently bind TEV, providing insight into the protease-trapping process. Bacterial A2Ms thus emulate critical initial steps of eukaryotic innate immune protection processes, suggesting that these enzymes are members of a rudimentary microbial immune system and play a role in bacterial protection from attack to their cellular integrity. Structure determination of Sa-A2M Sa-A2M is a single chain, 1,644 residue protein that includes an N-terminal 17 residue signal peptide and an LAGC lipobox. A clone expressing residues 19–1,644 of Sa-A2M with a 6xHis-tag and a thrombin site fused to the N terminus was expressed and purified, but only a single and irreproducible crystal was produced. We thus employed the surface entropy reduction approach [34] to search for patches of surface residues whose mutation could potentially promote local stability. Residues 98 and 99 were thus mutated into alanines. This variant labelled with selenomethionine was purified in the ‘native’ or preactivated form and produced crystals that diffracted X-rays to 2.95 Å. 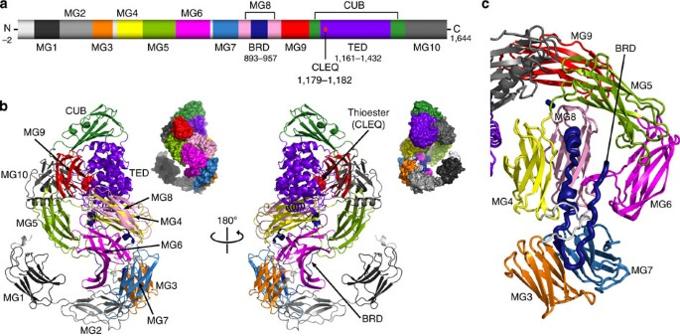Figure 1: Crystal structure ofS. typhimuriumalpha-2-macroglobulin (Sa-A2M). (a) Schematic of the 13 domains in Sa-A2M. The N-terminal 17-residue signal peptide and the LAGC lipobox sequence were absent in the clone used for crystallization. The domains are coloured identically ina–c. (b) The overall structure of Sa-A2M displayed is the preactivated form before reaction with proteases. The thioester site is buried in the interface between the TED and MG10 domains. MG1 and MG2 are only observed in bacterial A2Ms. MG1, normally anchored to the inner membranein vivo, is connected to MG2 by a flexible linker. (c) MG3–MG8 form a coiled arrangement that resembles a distorted key ring. The cavity formed by the key ring scaffold houses the partially observed bait region. The crystal structure of Sa-A2M was solved by performing a single-wavelength anomalous diffraction experiment at the European Synchrotron Radiation Facility (ESRF) in Grenoble, France ( Table 1 ). The crystal contained one molecule per asymmetric unit; the Lys98Ala/Lys99Ala mutations promoted crystal contacts between the backbone carbonyl of residue 101 and the side chain of residue 462 from a symmetry-related molecule ( Supplementary Fig. 1a ), which most probably stabilized the monomers enough to generate diffraction-quality crystals. Table 1 Data collection and refinement statistics. Full size table Model building of native Sa-A2M was challenging due to the large number of domains and the unexpected positions of macroglobulin-like domain (MG)1 and MG2. These two domains were found closely packed against other symmetry-related molecules, resulting in an intertwined configuration ( Supplementary Fig. 1b ). Subsequent to solving the structure of the native form of Sa-A2M, we solved the structure of a methylamine-treated form by incubating Sa-A2M with methylamine for 2 h at 20 °C before crystallization. Methylamine was present in both the crystallization and cryoprotectant-soaking steps to prevent reformation of the thioester. The structures of both the methylamine-treated Sa-A2M and a thioester pocket mutant (Tyr1175Gly) were solved by performing molecular replacement experiments using the structure of native Sa-A2M as a model. Crystal structure of Sa-A2M Sa-A2M is composed of 13 domains ( Fig. 1 ), all of which fold as variants of beta sandwiches with the exception of the TED, which consists of 14 alpha helices ( Fig. 1b ). Most of the beta sandwich domains appear to serve a structural role and are referred to as the MG domains. Residues 57–281 form MG1 and MG2, which are linked by a flexible loop. MG1 is the domain which is the farthest from the body of the structure; since the N terminus of Sa-A2M is expected to be anchored to the periplasmic inner membrane, as observed for ECAM [32] , MG1–MG2 could play the role of a linker associating the main body of Sa-A2M to the bilayer. Residues 282–1,010 fold into the six subsequent MG domains (MG 3–8), which together form 1.5 turns of a helical coil to generate what resembles a distorted ‘key ring’ ( Fig. 1c ) in an arrangement that is highly reminiscent of that of proteins of the eukaryotic A2M/complement/TEP superfamily. The key ring scaffold, also referred to as the beta-ring in TEP1 and complement C3, C4 and C5, provides a frame for a highly flexible stretch of amino acids in the bait region domain (BRD). The first half of the BRD extends from MG8 to MG3 and is adjacent to MG4 and MG7 on the concave side of the key ring scaffold. Interestingly, a segment of the BRD contributes one strand to the MG3 beta sheet before folding back towards MG8 through the key ring cavity. It is precisely this region that contains the bait site for protease cleavage (residues 925–950), and its high flexibility is evidenced from the fact that it can only be partly traced in the electron density map. Figure 1: Crystal structure of S. typhimurium alpha-2-macroglobulin (Sa-A2M). ( a ) Schematic of the 13 domains in Sa-A2M. The N-terminal 17-residue signal peptide and the LAGC lipobox sequence were absent in the clone used for crystallization. The domains are coloured identically in a – c . ( b ) The overall structure of Sa-A2M displayed is the preactivated form before reaction with proteases. The thioester site is buried in the interface between the TED and MG10 domains. MG1 and MG2 are only observed in bacterial A2Ms. MG1, normally anchored to the inner membrane in vivo , is connected to MG2 by a flexible linker. ( c ) MG3–MG8 form a coiled arrangement that resembles a distorted key ring. The cavity formed by the key ring scaffold houses the partially observed bait region. Full size image MG9 follows the key ring scaffold, and it is connected through the CUB (complement C1r/C1s, Uegf, Bmp1) domain to the TED domain. The TED domain is in a preactivated conformation that maintains the thioester site buried against MG10. In this conformation, it also interacts with MG4 and CUB, the latter of which is also connected at its C terminus to MG10. MG10 is markedly different from the other MG domains in that it has more beta strands and an alpha helix. The position of MG10 is stabilized by, in addition to other hydrogen bonds, the formation of a beta sheet with MG9. Notably, a hydrogen bond is observed between Tyr1626 of MG10 and Glu1181 of the thioester site in TED ( Supplementary Fig. 2 ) and could serve a local stabilizing role (see below). It is of note that MG10 is structurally reminiscent of the C-terminal, receptor-binding domain of eukaryotic alpha-macroglobulin [35] , [36] (r.m.s.d.=3.54 Å over 120 C-alpha atoms), but its involvement in protease clearance is to date unclear. Protection of the thioester by a tyrosine lock The thioester bond of Sa-A2M, which is formed between Cys1179 and Gln1182, is intact in the native structure ( Fig. 2a ) and buried between the TED and MG10 domains ( Fig. 2b ). Similarly to the structures of complement components C3, C4 and TEP1, the thioester site is found in a pocket surrounded by aromatic and hydrophobic residues. In Sa-A2M, the pocket is surrounded by Tyr1175, Tyr1177 and Trp1235 from the TED domain, as well as Met1625 and Tyr1626 from MG10. Notably, all of these residues are conserved in bacterial and eukaryotic A2M variants, with the exception of Tyr1175, which is present only in bacterial species ( Supplementary Fig. 3a ) and points directly towards the interior of the CXEQ pocket in the native structure ( Fig. 2 ). Despite being protected from hydrolysis by its location in the hydrophobic pocket, the thioester bond in Sa-A2M is located near the surface of the molecule ( Fig. 1b ). 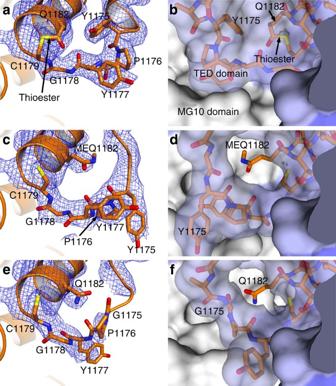Figure 2: Thioester site of Sa-A2M, methylamine-inactivated Sa-A2M and Sa-A2M Tyr1175Gly. (a), (c) and (e): The 2Fo-Fcelectron density contoured at 1 σ is shown. (b), (d) and (f): The surface representation is shown after rotating (a,c,f) ~180°. (a) In the untreated protein, a thioester bond between Cys1179 and Gln1182 is observed, as evidenced by the electron density connecting these two residues. (b) Before reaction with methylamine, the thioester, which is hidden from view, is buried between the TED and MG10 domain. Tyr1175 contributes to keeping the thioester buried and protected from hydrolysis. (c) Reaction with methylamine breaks the thioester bond between Cys1179 and Gln1182, and causes a conformational change of Tyr1175. (d) After the conformational change, the inactivated thioester is no longer buried in the TED domain. (e) Mutation of Tyr1175 to glycine results in loss of the thioester bond between Cys1179 and Gln1182. (f) Similarly to the methylamine-treated sample, the thioester in the Tyr1175Gly variant is no longer buried in the TED domain. Figure 2: Thioester site of Sa-A2M, methylamine-inactivated Sa-A2M and Sa-A2M Tyr1175Gly. ( a ), ( c ) and ( e ): The 2F o -F c electron density contoured at 1 σ is shown. ( b ), ( d ) and ( f ): The surface representation is shown after rotating ( a , c , f ) ~180°. ( a ) In the untreated protein, a thioester bond between Cys1179 and Gln1182 is observed, as evidenced by the electron density connecting these two residues. ( b ) Before reaction with methylamine, the thioester, which is hidden from view, is buried between the TED and MG10 domain. Tyr1175 contributes to keeping the thioester buried and protected from hydrolysis. ( c ) Reaction with methylamine breaks the thioester bond between Cys1179 and Gln1182, and causes a conformational change of Tyr1175. ( d ) After the conformational change, the inactivated thioester is no longer buried in the TED domain. ( e ) Mutation of Tyr1175 to glycine results in loss of the thioester bond between Cys1179 and Gln1182. ( f ) Similarly to the methylamine-treated sample, the thioester in the Tyr1175Gly variant is no longer buried in the TED domain. Full size image Previous studies with human and E. coli A2M have shown that reaction with methylamine inactivates the thioester and causes a major conformational change in the eukaryotic variant [5] , [19] , [32] , [33] , [37] , [38] , [39] . To address the issue of a potential conformational change in a bacterial A2M on activation, we solved the crystal structure of methylamine-treated Sa-A2M. Notably, the fold of methylamine-treated Sa-A2M is highly reminiscent of the native form, since it does not indicate any major differences in domain positions, and a structural alignment of the two molecules results in an r.m.s.d. of 0.35 Å (1,536 C-alpha atoms). Small-angle X-ray scattering (SAXS) experiments undertaken to explore potential conformational modifications on activation yielded curves that are nearly identical for native and methylamine-treated Sa-A2M ( Supplementary Fig. 4 ). These observations are thus supportive of fluorescence, analytical ultracentrifugation and native polyacrylamide gel electrophoresis (PAGE) studies of E. coli A2M that suggested that thioester cleavage did not lead to major conformational differences [32] , but differ from SAXS results obtained on the latter molecule, which indicated some degree of conformational modification on methylamine treatment [33] . Despite the fact that a major shift in domain positions could not be detected for Sa-A2M, reaction with methylamine caused cleavage of the thioester bond ( Fig. 2c ), causing Tyr1175 to be pushed away from the thioester site and the methylated Gln1182 to move towards its original position. Notably, Gln1182 is exposed to solvent when Tyr1175 is in the ‘open’ conformation ( Fig. 2d ). Since Tyr1175 is highly conserved among bacterial A2Ms and reaction with methylamine causes a drastic modification in its position, we postulated that this residue could be crucial for the formation and maintenance of the thioester bond ( Supplementary Fig. 3a ). To investigate thioester site stability in the absence of the Tyr1175 side chain, we solved the crystal structure of a Sa-A2M Tyr1175Gly point mutant. In this structure, the thioester bond is no longer shielded and is cleaved, potentially through hydrolysis by a water molecule from solvent, and Gln1182 moves into the position normally occupied by Tyr1175 ( Fig. 2e ). This observation strongly indicates that Tyr1175 is an essential component of a ‘locking mechanism’ that maintains the stability of the thioester bond in the native form. In the Tyr1175Gly variant, the electron density around residues 1,174–1,176 is weak, indicating that this region is more flexible. The flexibility of this loop removes its ability to protect the thioester site, and results in residue 1,182 becoming exposed to solvent ( Fig. 2f ), indicating that the lock is ‘open’. Mechanism of activation of Sa-A2M Following our discovery that methylamine treatment of Sa-A2M does not trigger a conformational change as it does in human A2M, we focused on deciphering the physiological mechanism of activation. In the native form of Sa-A2AM, the thioester site remains buried between the TED and MG10 domains. Cleavage at the bait site by a protease should activate Sa-A2M and trigger a conformational change by a yet undetermined mechanism that exposes the thioester site to the protease. However, in the crystal structure of Sa-A2M, the second half of the bait region is not observable due to the weak electron density for these flexible residues. The entire bait region could be observed to stretch across the concave pocket formed by the key ring scaffold after filling in the missing residues (939–955) using MODELLER ( Supplementary Fig. 5a ). Thus, to facilitate the investigation of the protease-trapping process after cleavage at the bait site, an artificial bait site for TEV protease was inserted into the centre of the bait region which, based on the structure of this model, should be easily accessible. Reaction products following proteolytic activation by TEV protease were characterized by mass spectrometry and denaturing gel electrophoresis. Sa-A2M containing the TEV-specific bait site (Sa-A2M-TB), methylamine-treated Sa-A2M-TB (Sa-A2M-TB-MA), native Sa-A2M and Sa-A2AM-TB Tyr1175Gly were incubated alone or with TEV at a molar ratio of 1:2 ( Fig. 3 , Table 2 ). Protease cleavage of Sa-A2M-TB at the bait region (residues 940/941) is expected to yield fragments of 102 kDa and 77 kDa, corresponding to the N-terminal fragment and the thioester-containing C-terminal fragment (CTF), respectively. Since TEV has a mass of 29 kDa, its covalent association to the TED domain is expected to yield a protease-bound C-terminal fragment (CTF-TEVP) of 106 kDa ( Fig. 3b ). This is confirmed both by SDS–PAGE ( Fig. 3a ) and mass spectrometry measurements ( Table 2 ). Interestingly, the CTF-TEVP band migrates anomalously and slower than expected. 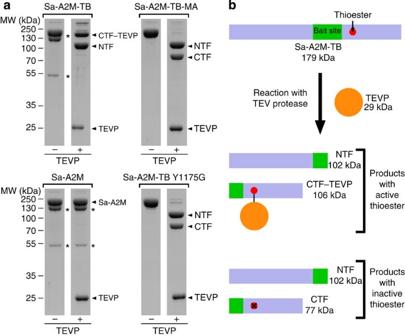Figure 3: TEV protease digestion profiles of Sa-A2M and Sa-A2M-TB. (a) In total, 40 μM of Sa-A2M-TB, Sa-A2M-TB-MA, Sa-A2M and Sa-A2M-TB Tyr1175Gly were incubated with 0 μM or 80 μM TEV protease. Reaction of TEV protease with Sa-A2M-TB and Sa-A2M-TB-MA shows the different products for samples with an active or inactive thioester, respectively. Sa-A2M without a TEV site is unaffected by the protease. TEV digestion of Sa-A2M-TB Tyr1175Gly resembles methylamine-treated Sa-A2M-TB, which indicates an inactive thioester. Heat degradation products (*) were observed in Sa-A2M-TB and Sa-A2M, a characteristic of samples with an active thioester. Such degradation products have also been observed in other thioester-containing proteins such as human A2M, C3 and C4, andE. coliA2M32,44,61. (b) A schematic diagram of the expected reaction products between TEV and Sa-A2M-TB with an active or inactive thioester. Figure 3: TEV protease digestion profiles of Sa-A2M and Sa-A2M-TB. ( a ) In total, 40 μM of Sa-A2M-TB, Sa-A2M-TB-MA, Sa-A2M and Sa-A2M-TB Tyr1175Gly were incubated with 0 μM or 80 μM TEV protease. Reaction of TEV protease with Sa-A2M-TB and Sa-A2M-TB-MA shows the different products for samples with an active or inactive thioester, respectively. Sa-A2M without a TEV site is unaffected by the protease. TEV digestion of Sa-A2M-TB Tyr1175Gly resembles methylamine-treated Sa-A2M-TB, which indicates an inactive thioester. Heat degradation products (*) were observed in Sa-A2M-TB and Sa-A2M, a characteristic of samples with an active thioester. Such degradation products have also been observed in other thioester-containing proteins such as human A2M, C3 and C4, and E. coli A2M [32] , [44] , [61] . ( b ) A schematic diagram of the expected reaction products between TEV and Sa-A2M-TB with an active or inactive thioester. Full size image Table 2 Electrospray ionisation–time of flight mass spectrometry analyses of reaction products between Sa-A2M variants and tobacco etch virus protease. Full size table Incubation of Sa-A2M-TB with methylamine before interaction with TEV should inactivate the thioester and preclude protease association. On incubation of a Sa-A2M-TB-MA with TEV, two bands of ~110 kDa and ~80 kDa are visualized on SDS–PAGE; mass spectrometry confirms that they correspond to N-terminal fragment and CTF without bound TEV ( Table 2 and Fig. 3a ). These observations thus confirm that in bacterial A2Ms, protease entrapment is also dependent on an intact thioester. To verify that the effects observed in the reactions of Sa-A2M-TB with TEV were caused by cleavage at the bait site, we incubated the protease with native Sa-A2M. As native Sa-A2M does not contain a TEV recognition site, cleavage products are not expected after reaction with the protease, which is what was observed ( Table 2 and Fig. 3a ). This confirms that cleavage at the bait site must occur prior to covalent linkage of TEV by Sa-A2M, even when the thioester is intact. The crystal structure of the Sa-A2M Tyr1175Gly variant (described above) shows that the thioester site is disrupted by the Tyr1175Gly mutation. Sa-A2M-TB Tyr1175Gly was thus incubated with TEV to examine the effects of this mutation on its activity. Two major bands, corresponding to the N-terminal and C-terminal regions of the molecule, appear after digestion, similarly to those identified on reacting TEV with Sa-A2M-TB-MA ( Table 2 and Fig. 3a ). This indicates that, as predicted from the crystal structure of Sa-A2M Tyr1175Gly, Tyr1175 is a key element of the locking mechanism which protects the thioester from hydrolysis; its mutation to glycine inactivates the thioester, preventing TEV from covalently binding Sa-A2M even in the presence of a TEV-specific bait region. A2Ms are hallmarks of the eukaryotic innate immunity system, and until recently, had been believed to exist uniquely in metazoans. The identification of genes encoding A2M-like proteins in genomes of a variety of pathogenic bacteria and eukaryotic-colonizing organisms, suggested to have occurred through horizontal gene transfer from eukaryotes to prokaryotes, indicated that inactivation of a large spectrum of exoproteases could play key roles during the infectious or surface colonization processes [28] , [32] . Eleven of the 13 domains in the structure of Sa-A2M reported here resemble those in the other proteins of the A2M/complement/TEP superfamily ( Fig. 4 ). Sa-A2M contains two hallmark features of an A2M: a thioester site and a bait region. Sa-A2M does not have the anaphylatoxin or C-terminal C345C domains that are found in complement proteins, and is structurally more similar to A2M. Therefore, its mechanism of activation is also more analogous to that of eukaryotic A2Ms, and occurs through proteolytic cleavage at the bait site. This is in contrast to complement C3 where activation occurs through cleavage and removal of the anaphylatoxin domain. 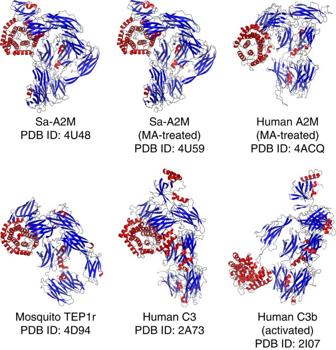Figure 4: Structural comparison of Sa-A2M and related structures. The structures of Sa-A2M, methylamine-treated Sa-A2M, methylamine-treated human A2M, mosquito TEP1r, human complement C3 and activated human complement C3b are shown as representatives of related structures in the A2M family that are currently available. They are coloured according to secondary structure, where the alpha helices, beta sheets and loops are coloured red, blue and grey, respectively. Notably, the structures of complement C3 and complement C3b demonstrate the large movements that the TED domain can undergo after activation by a proteolytic event. Figure 4: Structural comparison of Sa-A2M and related structures. The structures of Sa-A2M, methylamine-treated Sa-A2M, methylamine-treated human A2M, mosquito TEP1r, human complement C3 and activated human complement C3b are shown as representatives of related structures in the A2M family that are currently available. They are coloured according to secondary structure, where the alpha helices, beta sheets and loops are coloured red, blue and grey, respectively. Notably, the structures of complement C3 and complement C3b demonstrate the large movements that the TED domain can undergo after activation by a proteolytic event. Full size image Strikingly, in addition to displaying a multidomain architecture and the hallmark features of eukaryotic A2Ms, Sa-A2M harbours the MG1 and MG2 domains, which are unique to bacterial A2Ms. Since the N terminus of Sa-A2M is anchored to the inner membrane of the bacterium, these two additional domains may impart Sa-A2M with more freedom of motion and range for trapping proteases and/or provide additional shielding of the trapped protease from its substrates. This may be an adaptation arising from the localization of bacterial A2Ms to the cell wall in contrast to eukaryotic A2M/complement/TEP proteins, which are found in the circulatory system. The structural alignment of the available structures from the A2M/complement/TEP superfamily also provides insight into the catalytic activity of Sa-A2M. In the complement cascade, after activation of C3, a histidyl residue converts the thioester to an acyl-imidazole intermediate and a thiolate anion. This causes the thioester of activated C3b to favour binding to hydroxyl groups rather than amines, which makes it more reactive towards water and carbohydrates [40] , [41] . This histidyl residue is also present in bovine C3, mosquito TEP1, CD109, A2ML1 and the archaeal A2M-like proteins of Methanococcoides burtonii and Methanolobus psychrophilus R15, but is absent from Sa-A2M. Thus, bacterial A2Ms are expected to exhibit higher activity towards lysine groups, as is the case for human A2M [42] , [43] . Consequently, Sa-A2M has a longer opportunity after activation to trap a protease before the thioester becomes inactivated by hydrolysis. The crystal structure of Sa-A2M shows strong density in the thioester site, which confirms that even though Sa-A2M harbours a leucine within the thioester motif (CLEQ) instead of a glycine (CGEQ) as in other A2M-like proteins, the thioester site is stably formed ( Fig. 2a ). Structural alignment of the thioester pockets for Sa-A2M and human complement C3, bovine complement C3, human complement C4 and mosquito TEP1 ( Fig. 5 ) reveal that all are formed by aromatic and hydrophobic residues that shield the thioester from hydrolysis. The tyrosyl residues equivalent to Tyr1626 of Sa-A2M are observed in all aforementioned eukaryotic A2M/complement-like proteins and form a hydrogen bond with the glutamyl residue of the CXEQ motif ( Fig. 5 , Supplementary Figs 2 and 3 ) and thus could serve as an anchor that aids in stabilizing the site. Some of the other amino acids in the pocket of Sa-A2M are positioned slightly differently from the other proteins, but achieve the same effect of blocking out solvent, thus demonstrating that protection of the thioester site before activation is a common requirement in the A2M/complement/TEP proteins. More specifically, Tyr1175 and Tyr1177 of Sa-A2M, which are located adjacent to the thioester, appear to occupy similar spaces as Tyr1559 and Tyr1525 of complement C4A, which are located on the MG8 domain (equivalent to MG10 of Sa-A2M). Met1625 of Sa-A2M and Met1483 of C4A also display small differences in their side-chain locations. Sequence alignment of bacterial A2Ms and other A2M-like proteins show that the thioester pocket residues are highly conserved within their own subfamily ( Supplementary Fig. 3 ). 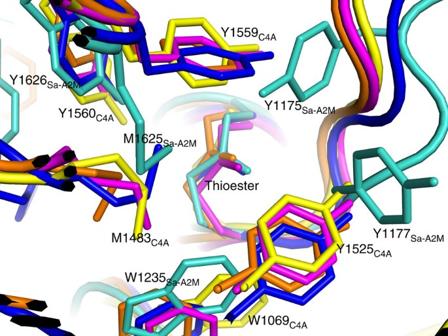Figure 5: Structural alignment of thioester sites of A2M-like proteins. The thioester sites of the A2M-like proteins are surrounded by aromatic and hydrophobic residues. For clarity, only the thioesters and the surrounding aromatic and methionyl residues are shown. Structural alignment reveals that the thioester pockets of human complement C3 (magenta, 2A73), bovine complement C3 (orange, 2B39), human complement C4 (yellow, 4FXK), mosquito TEP1 (blue, 4D94) and Sa-A2M (turquoise) are similar in that the thioesters are shielded from the solvent. Interestingly, the thioester pocket of Sa-A2M is formed by amino-acid types similar to those in other A2M-like proteins, but has a unique configuration. Figure 5: Structural alignment of thioester sites of A2M-like proteins. The thioester sites of the A2M-like proteins are surrounded by aromatic and hydrophobic residues. For clarity, only the thioesters and the surrounding aromatic and methionyl residues are shown. Structural alignment reveals that the thioester pockets of human complement C3 (magenta, 2A73), bovine complement C3 (orange, 2B39), human complement C4 (yellow, 4FXK), mosquito TEP1 (blue, 4D94) and Sa-A2M (turquoise) are similar in that the thioesters are shielded from the solvent. Interestingly, the thioester pocket of Sa-A2M is formed by amino-acid types similar to those in other A2M-like proteins, but has a unique configuration. Full size image Proteins containing the CXEQ motif are known to become cleaved between the glutamyl and glutaminyl residues of the CXEQ thioester motif when denatured by SDS–PAGE [41] , [44] . For Sa-A2M-TB and Sa-A2M, this cleavage produced two fragments of ~130 kDa and ~55 kDa ( Fig. 4a ). These cleavage products were not visible for Sa-A2M-TB-MA or Sa-A2M-TB Tyr1175Gly, confirming the loss of the thioester bond in these samples. All the expected products following TEV protease reaction migrated in SDS–PAGE in positions that corresponded to the expected mass spectrometry value, except for the CTF of Sa-A2M-TB covalently bound to TEV, which migrated as a ~150-kDa fragment by SDS–PAGE instead of at the expected size of 106 kDa. The anomalous migration is likely a result of the non-linearity of the fragment, a consequence of the position of the covalent bond between the thioester in Sa-A2M-TB and TEV. A2M from E. coli was shown to block large macromolecules from accessing a trapped protease [32] , and we show here that this trapping process involves activation of the thioester by cleavage at the bait region. Thus, we would like to suggest a model for protease entrapment by A2M in that after proteolytic cleavage at the bait region, the positions of the TED, CUB and MG10 domains are altered causing the TED domain to shift towards the protease, allowing the thioester to covalently bind it ( Supplementary Fig. 5b ). The domain rearrangements in A2M should be less drastic than those observed for C3 considering the relative position of the protease. In the trapped conformation, the position of the protease remains fixed so that the walls of the A2M, which is monomeric and does not benefit from the cage-like architecture of eukaryotic A2Ms, can partially shield it from its substrates. We hypothesize that the trapped conformation is relatively fixed, as a flexible system would be less efficient in preventing the active site of the protease from becoming exposed. Further studies with the Sa-A2M-TB variant that stably traps target proteases may shed more light on this topic. In summary, our findings reveal that bacterial A2Ms are novel members of the A2M/complement/TEP superfamily, all of which are known to play a role in the innate immune system of eukaryotes. In bacteria, A2Ms were proposed to act by providing general defence of the periplasm against proteases secreted by attacking organisms. In addition to conferring protection from host proteases during the infectious process, bacterial A2Ms might also inhibit endopeptidases of competing bacteria or phages. Our findings suggest that bacterial A2Ms are representatives of a rudimentary immune system evolved to mimic initial key steps of the eukaryotic innate immune pathway. DNA cloning and protein purification of Sa-A2M STM2532 , the gene for A2M from Salmonella enterica serovar Typhimurium strain LT2, was amplified using PCR and cloned into the pET28a vector (Novagen) using the Nde I and Xho I sites ( Supplementary Table 1 ). The 18 residues at the N terminus, which include the signal sequence and the cysteine that becomes palmitoylated, were removed. The resulting construct encoded an N-terminal 6xHis-tag and a thrombin cleavage site, MGSSHHHHHHSSGLVPRGSHM, followed by residues 19–1,644 of Sa-A2M. Escherichia coli BL21(DE3) cells containing the expression vector were grown in LB media containing 50 μg ml −1 kanamycin at 37 °C until the OD at 600 nm reached 0.6–0.7 before induction of protein expression by the addition of 1 mM isopropyl β- D -thiogalactopyranoside. Protein expression continued overnight for approximately 16 h at 25 °C. Cells were harvested by centrifugation at 5,500 g for 20 min at 4 °C and resuspended in buffer A (50 mM HEPES pH 7.5, 200 mM NaCl) supplemented with 0.7 μg ml −1 antiproteases aprotinin, 0.5 μg ml −1 leupeptin, 0.7 μg ml −1 pepstatin and 1 mM phenylmethyl sulphonyl fluoride. Cells were lysed by sonication before removal of cell debris by centrifugation at 39,000 g for 45 min at 4 °C. All purification steps were carried out at 4 °C. The cell extract was supplemented with 5 mM imidazole and loaded onto a HisTrap FF column (GE Healthcare). The protein was eluted with a linear gradient to 0.5 M imidazole, and the fractions containing Sa-A2M were pooled and dialyzed overnight against 50 mM HEPES pH 8 using a dialysis membrane with a molecular-weight cutoffs of 50 kDa (Spectrum Laboratories). Sa-A2M was loaded onto a Resource Q anion-exchange column (GE Healthcare) and eluted with a linear gradient to 50 mM HEPES pH 8, 0.5 M NaCl. The fractions containing Sa-A2M were pooled and concentrated using Vivaspin centrifugal filters (Sartorius) before loading onto a Superdex 200 gel filtration column (GE Healthcare) equilibrated with buffer A. The central fractions of the peak containing Sa-A2M were pooled, concentrated and exchanged into the appropriate buffer using centrifugal filtration. Protein concentration was measured with a NanoDrop 2000c (Thermo Scientific) using an extinction coefficient at 280 nm of 229,070 M −1 cm −1 , as calculated by the ExPASy ProtParam tool. The same E. coli strain and expression vector that was used for expressing native protein were also used for selenomethionine incorporation. Selenomethionine-labelled protein was produced by the methionine pathway inhibition method and purified using the same protocol as for the native protein [45] , [46] , [47] . Crystallization and structure determination Lysines at position 98 and 99 were mutated to alanines, as suggested by the Surface Entropy Reduction prediction server [48] , using site-directed mutagenesis to promote protein crystallization ( Supplementary Table 1 ). Crystallization conditions were found by using the High Throughput Crystallization Laboratory at the Partnership for Structural Biology in Grenoble [49] . Initial crystallization conditions identified contained 0.02 M CaCl 2 , 0.1 M sodium acetate pH 4.6, 15% 2-methyl-2,4-pentanediol; 0.1 M sodium acetate pH 4.6, 4% PEG 4000; 0.1 M citric acid pH 4, 10% PEG MME 5000; or 0.1 M NaCl, 0.1 M sodium acetate pH 4.6, 12% isopropanol. In order to grow larger crystals, the Sa-A2M Lys98Ala/Lys99Ala variant was crystallized by hanging drop vapour diffusion by mixing equal volumes of 10 mg ml −1 Sa-A2M Lys98Ala/Lys99Ala with the crystallization solution of 0.1 M sodium acetate pH 5.2, 4% PEG 4000. Crystals were grown at 4 °C and appeared within 1 week. Selenomethionine-substituted crystals were grown in the same condition utilizing streak seeding with native crystals. Crystals were cryoprotected by successively soaking them for 10 s and 5 s in the crystallization solutions containing 15% and 30% glycerol, respectively, before flash-cooling in liquid nitrogen. For the methylamine-treated structure, 5 μM Sa-A2M Lys98Ala/Lys99Ala was incubated in buffer A, 0.5 M methylamine at 20 °C for 2 h. After the reaction, the protein was concentrated to 10 mg ml −1 using a centrifugal filter and exchanged into 20 mM HEPES pH 7.5, 10 mM NaCl and 0.5 M methylamine. The methylamine-treated Sa-A2M Lys98Ala/Lys99Ala was crystallized in 0.1 M sodium acetate pH 5.2, 7% PEG 4000 without seeding. Crystals were cryoprotected by successively soaking for 2 min, 2 min, 2 min and 5 min in 0.1 M sodium acetate pH 5.2, 7% PEG 4000, 0.5 M methylamine containing 0%, 10%, 20% and 30% glycerol, respectively, before flash-cooling in liquid nitrogen. The Sa-A2M Lys98Ala/Lys99Ala/Tyr1175Gly variant was crystallized by mixing 20 mg ml −1 protein with 0.1 M sodium acetate pH 4.8, 2.5% PEG 4000. The crystals were cryoprotected by successively soaking for 10 s, 10 s and 5 s in the crystallization condition containing 10%, 20% and 30% glycerol, respectively, before flash-cooling in liquid nitrogen. A data set was collected at 100 K from a crystal of SeMet-substituted Sa-A2M Lys98Ala/Lys99Ala at the selenium K edge ( λ =0.97939 Å) on the ID29 beamline of the ESRF (Grenoble, France), which was equipped with a Pilatus 6M detector. A data set for methylamine-treated Sa-A2M Lys98Ala/Lys99Ala was collected at the ID23-2 beamline ( λ =0.8726 Å) of the ESRF, which was equipped with a Mar225 detector. A data set for the Sa-A2M Lys98Ala/Lys99Ala/Tyr1175Gly variant was collected on ID29. Diffraction data were indexed, integrated and scaled using the XDS program package [50] . The untreated SeMet-substituted Sa-A2M Lys98Ala/Lys99Ala was solved by single-wavelength anomalous diffraction phasing using AutoSol and AutoBuild from the PHENIX suite to automatically find the selenium sites, phase and build the structure [51] . Structures for the methylamine-treated protein and the Tyr1175Gly variant were solved by molecular replacement with Phaser using the structure of the untreated protein as the search model [52] . Cycles of refinement and manual building were performed using Phenix.Refine and Coot, respectively [51] , [53] ( Supplementary Fig. 6 ). A riding hydrogen model was used during refinement. The Ramachandran plot for Sa-A2M Lys98Ala/Lys99Ala, methylamine-treated Sa-A2M Lys98Ala/Lys99Ala and Sa-A2M Lys98Ala/Lys99Ala/Tyr1175Gly showed 91%, 90% and 90% of the residues in the most favoured regions, respectively, and 1.8%, 2.2% and 2.9% outliers, respectively. PyMOL was used to create the structural figures ( http://www.pymol.org/ ). SAXS X-ray scattering data were collected for the untreated and methylamine-treated Sa-A2M on the BM29 beamline of the ESRF, which was equipped with a Pilatus 1-M detector ( s =4 π sin θ / λ where 2 θ is the scattering angle and λ =0.992 Å). Methylamine-treated Sa-A2M was prepared by incubating 5 μM of Sa-A2M with buffer A, 0.5 M methylamine at 20 °C for 2 h followed by purification with a Superdex 200 column equilibrated in buffer A. Both the untreated and methylamine-treated Sa-A2M samples were exchanged into buffer A, 2 mM dithiothreitol using centrifugal filtration devices, and the filtrates were used for background subtraction. Bovine serum albumin (4.05 mg ml −1 ) was measured for calibration, and the molecular weight of Sa-A2M was calculated by comparison of the forward intensities at zero angle (I(0)). Scattering data were collected for a concentration gradient of 9.04 mg ml −1 , 4.52 mg ml −1 , 2.26 mg ml −1 and 1.13 mg ml −1 for untreated Sa-A2M and 9.13 mg ml −1 , 4.56 mg ml −1 , 2.28 mg ml −1 and 1.14 mg ml −1 for methylamine-treated Sa-A2M. Ten 1-s exposure frames were collected at 20 °C for each sample in flow-mode with 90 μl of sample [54] . Repulsive interparticle effects were observed, and the data were extrapolated to infinite dilution using ALMERGE [55] . R g and I(0) were estimated automatically by Guinier analysis using AUTORG [56] . DATGNOM was used to automatically estimate the D max and calculate the distance distribution function [56] . CRYSOL was used to calculate the theoretical fitting curve from the crystal structure of Sa-A2M [57] . Artificial TEV protease bait site An artificial TEV protease cleavage site was introduced into Sa-A2M in order to use TEV as a model protease. For these experiments, the N-terminal 6xHis-tag and thrombin cleavage site were removed, and a C-terminal 6xHis-tag, LEHHHHHH, was added by using PCR amplification and cleavage/ligation into the Nco I and Xho I sites of pET28a ( Supplementary Table 1 ). The amino-acid sequence ENLYFQG was substituted into the bait site (residues 935–941) by using site-directed mutagenesis ( Supplementary Table 1 ). The partially missing bait region was visualized by filling in the missing residues using the Chimera interface for MODELLER [58] , [59] . The binding of TEV protease was visualized by manually docking it next to the TEV protease cleavage site [60] . In total, 40 μM Sa-A2M-TB, Sa-A2M-TB-MA, Sa-A2M and Sa-A2M-TB Y1175G were reacted with 0 μM and 80 μM TEV protease in buffer A, 1 mM dithiothreitol, 0.5 mM EDTA overnight at 4 °C. For methylamine-treated samples, 67 μM Sa-A2M was incubated with buffer A, 0.33 M methylamine at 20 °C for 10 min before incubating with TEV protease. Final concentration of methylamine in the TEV protease reaction was 0.2 M. The reaction products of TEV protease and Sa-A2M were analysed by electrospray ionisation–time of flight mass spectrometry and SDS–PAGE. For SDS–PAGE, the samples were prepared by mixing with Laemmli sample buffer and heating to 98 °C for 5 min. How to cite this article: Wong, S. G. et al . Structure of a bacterial α 2 -macroglobulin reveals mimicry of eukaryotic innate immunity. Nat. Commun. 5:4917 doi: 10.1038/ncomms5917 (2014). Accession codes : The coordinates and structure factors have been deposited in the Protein Data Bank under the accession codes 4U48 , 4U59 , and 4U4J for the native, methylamine-reacted, and mutated forms of Sa-A2M, respectively.